Licensing MLH1 sites for crossover during meiosis During meiosis, homologous chromosomes synapse and recombine at sites marked by the binding of the mismatch repair protein MLH1. In hexaploid wheat, the Ph1 locus has a major effect on whether crossover occurs between homologues or between related homoeologues. Here we report that—in wheat–rye hybrids where homologues are absent— Ph1 affects neither the level of synapsis nor the number of MLH1. Thus in the case of wheat–wild relative hybrids, Ph1 must affect whether MLH1 sites are able to progress to crossover. The observed level of synapsis implies that Ph1 functions to promote homologue pairing rather than suppress homoeologue pairing in wheat. Therefore, Ph1 stabilises polyploidy in wheat by both promoting homologue pairing and preventing MLH1 sites from becoming crossovers on paired homoeologues during meiosis. During meiosis, homologous chromosomes are synapsed along their length by the loading of a proteinaceous structure, the synaptonemal complex, between them [1] . Within this framework, homologues can recombine. When the synaptonemal complex is degraded, crossovers (COs) or chiasmata enable the homologues to remain associated at metaphase I and so segregate properly [1] . Two classes of COs coexist in plants [2] . Class I gives rise to interfering COs and is thought to constitute the main pathway in plants [2] . Class II results in non-interfering COs [3] . Class I COs require MLH1, a DNA mismatch repair protein, part of the MutL complex, that is required for resolution of Double Holliday Junctions as COs, but not as non-crossovers (NCO). In all mammalian and diploid plant species so far studied, the presence of MLH1 sites on paired chromosomes at diplotene is the final marker for sites that will result in COs [4] , [5] . Despite possessing three related genomes (A, B and D), hexaploid wheat (2n=42) behaves as a diploid at meiosis. The major regulator of homoeologue pairing and recombination in wheat, the Ph1 locus [6] , ensures that recombination is restricted to true homologues rather than homoeologues (equivalent chromosomes from other genomes) [7] . A number of studies have analysed Ph1 ’s effect on chromosome organisation in premeiotic and early meiotic stages [8] , [9] , [10] , [11] . Here we study the dynamics of synapsis and the loading of the recombination machinery, and assess whether the formation and progression of these events are affected by the presence of Ph1 . In wheat, whether the Ph1 is present or not, the overall level of synapsis is similar; however, significant homoeologous synapsis occurs at late pachytene in the absence of Ph1 (ref. 7 ). This synapsis may or may not result in chiasmata, as univalent, bivalents and multivalents are observed at metaphase I. The number of MLH1 sites on paired chromosomes during diplotene marks sites that will become interfering COs. It has been shown in wheat that the distribution and frequency of COs between homologues and homoeologues are similar in the absence of Ph1 (ref. 12 ), suggesting that this locus is affecting the major class I interfering pathway dependent on the MLH1 protein. Thus the number of MLH1 sites would be expected to depend on the presence or absence of Ph1. Wheat has normally at least one chiasma linking each of the arms of the 21 homologue pairs in the presence of Ph1 . So about 42 MLH1 sites would be expected to be present in diplotene meiocytes. Consistent with this prediction, 48±4 MLH1 sites are observed in the presence of Ph1 ( Fig. 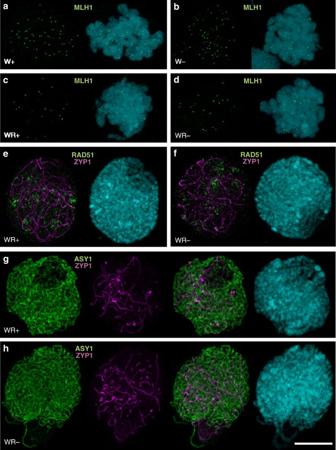Figure 1: Immunolocalization of meiotic proteins in wheat (W) and wheat–rye hybrids (WR) meiocytes in the presence (+) and absence (−) of thePh1locus. MLH1 (green) at diplotene in wheatPh1+(a), wheatPh1−(b), wheat–ryePh1+(c) and wheat–ryePh1−(d). RAD51 (green) and ZYP1 (magenta) at zygotene in wheat–ryePh1+(e) and wheat–ryePh1−(f). ASY1 (green) and ZYP1 (magenta) at zygotene in wheat–ryePh1+(g) and wheat–ryePh1−(h). DAPI staining in blue. Scale bar, 10 μm. 1a ; Table 1 ). When Ph1 is absent, on average seven chromosome arms lacked chiasmata at metaphase I ( Supplementary Table 1 ). Consequently, fewer MLH1 sites would be expected. However, surprisingly, the number of MLH1 sites is not decreased (52±5 at diplotene; Fig. 1b ; Table 1 ). This indicates that in the absence of Ph1 , when both homologous and homoeologous synapsis occurs [7] , the number of COs does not correspond with the number of MLH1 sites. The presence of slightly more MLH1 sites (48) than COs (42) may be because some of the MLH1 sites are on homoeologous chromosomes which would not progress to COs. The fact that we observe about 50 MLH1 sites in both the presence and absence of the Ph1 locus suggests some kind of homeostatic control to maintain CO number as has been reported in yeast, worms and mammals [13] . Figure 1: Immunolocalization of meiotic proteins in wheat (W) and wheat–rye hybrids (WR) meiocytes in the presence (+) and absence (−) of the Ph1 locus. MLH1 (green) at diplotene in wheat Ph1+ ( a ), wheat Ph1− ( b ), wheat–rye Ph1+ ( c ) and wheat–rye Ph1− ( d ). RAD51 (green) and ZYP1 (magenta) at zygotene in wheat–rye Ph1+ ( e ) and wheat–rye Ph1− ( f ). ASY1 (green) and ZYP1 (magenta) at zygotene in wheat–rye Ph1+ ( g ) and wheat–rye Ph1− ( h ). DAPI staining in blue. Scale bar, 10 μm. Full size image Table 1 Number of MLH1 foci and synaptonemal complex measurements. Full size table The effect of homoeologous synapsis on the number of MLH1 sites can be studied more directly in a situation where no homologous synapsis can occur. Wheat–rye hybrids contain a haploid set of 21 wheat chromosomes and a haploid set of seven rye chromosomes, thus possessing 28 homoeologues but no homologues. Several studies have reported an average of less than one rod bivalent in these hybrids, implying one chiasma or less at metaphase I with Ph1 present ( Supplementary Fig. 1 ). In contrast, an average of 7.8 rod bivalents or more than 15 chromosome arms are linked by chiasmata in the absence of Ph1 ( Supplementary Fig. 1 ). Thus it would be reasonable to expect only one MLH1 site in the presence of Ph1 but around 7 or 8 MLH1 sites in its absence. Again surprisingly, similar numbers of MLH1 sites are observed at diplotene whether in the presence or absence of Ph1 (19±3 and 22±3, respectively; Fig. 1c,d ). Therefore we can confirm that the number of MLH1 sites does not correlate directly with the number of COs when homoeologous synapsis occurs; only when homologues synapse. It is known that there are several fold more double-strand breaks generated at the start of meiosis, than are processed later into COs, and that there is a significant level of double-strand break repair using sister chromatids during meiosis [14] . In fact it has been reported that about a third of all double-strand breaks might be repaired using sister chromatids during meiosis [15] . Although our results show more MLH1 sites than would be expected from the number of COs with Ph1 either present or absent, if these MLH1 sites included sister chromatid repair sites, there would be substantially more than the number observed. Haploid Arabidopsis exhibits little synapsis and no chromosome fragmentation at metaphase I [16] , implying that double-strand breaks have been repaired using sister chromatids. However there is only an average of one MLH1 site observed at diplotene in this haploid [16] , indicating that MLH1 is not marking the sites of sister chromatid repair. Therefore, although we do observe more MLH1 sites than COs, the vast majority of MLH1 sites in the wheat–rye hybrid must mark Double Holliday Junctions between homoeologues that fail to be processed into COs after MLH1 loading, and then are processed into NCOs as the synaptonemal complex is degraded. Interestingly, deleting Ph1 does alleviate to some extent the stalling of MLH1 sites, as seven to eight of these sites managed to progress further and crossover. Molecular analysis of the Ph1 locus revealed that it carries a cluster of defective kinases [17] , [18] ; and indeed, the closest homologue of the Ph1 kinase in Arabidopsis also regulates pairing and recombination [19] . Proteomic analysis showed that deletion of Ph1 leads to increased phosphorylation at Cdk2-type sites during meiosis [18] , which implies that the presence of Ph1 decreases Cdk2-type phosphorylation. Consistent with this, treatment with okadaic acid, an inhibitor of phosphatase activity, increases Cdk2-type phosphorylation, and phenocopies the deletion of Ph1 by inducing COs [20] . Thus deleting Ph1 or treating with okadaic acid, both of which increase Cdk2-type activity, lead to an increased efficiency in processing of MLH1 sites on paired homoeologues into COs. Consistent with these observations, studies indicate that the MLH1 complex in mouse associates with Cdk2 on Double Holliday Junctions [4] , and that there is a requirement for Cdk activity in the resolution of the junction between homologues as a CO in Caenorhabditis elegans [21] . The level of homoeologue synapsis is reduced by the presence of Ph1 (ref. 7 ). However we have shown that there are similar numbers of MLH1 sites in either the presence or absence of Ph1. This implies that in the wheat–rye hybrid, where only homoeologues are present, Ph1 might not have a major effect on earlier meiotic pairing events as has been shown in wheat. To assess whether this is indeed the case, we used an antibody against RAD51, which marks sites of double-strand break formation, to assess the number of sites and their processing dynamics during earlier meiosis with and without Ph1 . In both cases, the RAD51 sites are observed early in leptotene, increase during zygotene ( Fig. 1e,f ) and disappear later in meiosis when Double Holliday Junctions are formed. The numbers of RAD51 sites observed in wheat–rye meiocytes, along with their dynamics, are indeed similar in hybrids with and without Ph1 . ASY1 is part of the lateral element of the synaptonemal complex around which each chromosome, comprising two sister chromatids, is organized; whereas the ZYP1 is part of the central region, which assembles between the lateral elements. The comparisons of the total lengths of the ZYP1-labelled elements with those of the ASY1, provides an indication of the level of synapsis achieved at pachytene when the synaptonemal complex is established ( Fig. 1g,h ; Table 1 ). The average total length of ASY1 elements traced at pachytene is 1,594±540 μm with Ph1 , and 1,662±535 μm without Ph1 ; and for ZYP1 elements, 403±89 μm with Ph1 and 378±141 μm without Ph1 . The level of overall synapsis is 27%±9 with Ph1 and 26%±15 without Ph1, indicating no significant difference. During this analysis, some synapsed bivalents could be traced almost in their entirety in the wheat–rye hybrids. The level of synapsis, the occurrence of synapsed bivalents, the rye genome structure [22] and the number of MLH1 sites are all consistent with reported preferential chiasma formation between the A and the D genomes in the wheat–rye hybrid in the absence of Ph1 (ref. 23 ). Potentially 14 of the 28 homoeologues could preferentially synapse with at least one MLH1 site per paired arm, resulting in a minimum of 14 MLH1 sites. Surprisingly, homoeologue synapsis is not reduced at pachytene in the hybrid, as it is in wheat itself, by the presence of Ph1 (ref. 7 ). The hybrid possesses just homoeologues, whereas wheat possesses both homologues and homoeologues. Suppression of homoeologue synapsis therefore requires the presence of both homologues as well as Ph1 . This implies that Ph1 promotes homologue pairing, rather than suppressing homoeologue pairing, as homoeologue pairing during pachytene occurs in the hybrid even in the presence of Ph1 . The presence of homologues has been shown to trigger chromosome elongation events on both homologues as part of the initial pairing process in wheat and C. elegans [10] , [24] . This elongation event is initiated in the telomere regions in wheat [10] . Ph1 affects telomere dynamics [25] , as well as synchronization of the elongation events at the onset of meiosis. Cdk2 colocalizes with MLH1 on the paired chromosomes and to the telomere regions affecting their dynamics during mouse meiosis [26] . Therefore it is conceivable that the promotion of homologous synapsis in wheat by Ph1 may simply be through a Cdk effect on the telomere regions. Thus Ph1 stabilizes wheat as a polyploid during meiosis by both promoting homologue pairing in early meiosis and preventing MLH1 sites on paired homoeologues from becoming COs later in meiosis. In the case of wheat–wild relative hybrids used by breeders to introduce important traits from relatives, Ph1 suppresses recombination between homoeologues by just preventing the MLH1 sites becoming COs. Plant material The tillers used for this study came from hexaploid wheat ( Triticum aestivum cv Chinese Spring (CS)) and crosses between rye ( Secale cereale cv Petkus) and hexaploid wheat (CS) either carrying or lacking the Ph1 locus ( ph1b deletion) [27] . Seeds were germinated on Petri dishes for 3 to 4 days. The seedlings were vernalized for 3 weeks at 5 °C and then transferred to a controlled-environment room until meiosis with the following growth conditions: 16 h light/8 h night photoperiod at 20 °C day and 15 °C night, with 70% humidity. Plants were collected after 6 to 7 weeks for meiosis studies. Meiosis staging and polyacrylamide embedding of meiocytes Meiocytes of wheat and wheat–rye hybrids were embedded in acrylamide to preserve their three-dimensional (3D) architecture. Embedding of meiocytes was based upon the method of Bass et al. [28] Briefly, tillers were harvested when the flag leaf was starting to emerge (around 2 cm). For each dissected floret, one of the three synchronized anthers was squashed in acetocarmine stain and examined under the light microscope to identify the appropriate stage of meiosis. The two remaining anthers were harvested into buffer A (15 mM Pipes-NaOH pH 6.8, 80 mM KCl, 20 mM NaCl, 0.5 mM EGTA, 2 mM EDTA, 0.2 mM spermine tetra HCl, 0.5 mM spermidine, 1 mM DTT, 0.32 M sorbitol) and the anthers from several plants were pooled. Anthers were then fixed in freshly prepared 4% paraformaldehyde for 15 min and washed twice in buffer A for 10 min. Anthers were macerated in buffer A and the meiocyte suspension was used to prepare the polyacrylamide pads. 10 μl of the meiocyte suspension were transferred onto a coverslip (24 × 24 mm) followed by immediate addition of 5 μl of activated acrylamide stock. The activated acrylamide stock was made by addition of 5 μl of 20% ammonium persulphate and 5 μl of 20% sodium sulphite to 100 μl of acrylamide stock (50 μl 2 × buffer A, 50 μl 30% 29:1 acrylamide/bis-acrylamide). The polymerising suspension was covered by another coverslip positioned with an overhang to allow easy removal after polymerisation. The coverslip was removed after 1 h, leaving a thin pad of acrylamide with embedded meiocytes attached to the slide. All washing steps below consisted of placing 2 ml on top of the face-up acrylamide placed in a petri dish (40 × 40 mm). Solutions were carefully removed by aspiration to avoid disturbing the acrylamide pads. Immunolocalization of meiotic proteins The meiotic nuclei embedded in polyacrylamide were washed twice in buffer A for 10 min to remove unpolymerized acrylamide, followed by 1-h wash in phosphate-buffered saline (PBS), 1% Triton X-100, 1 mM EDTA pH 8 and 2-h incubation in blocking buffer (3% BSA in PBS, 0.1% Tween 20, 1 mM EDTA pH 8). Acrylamide pads were incubated with the appropriate antibodies diluted 1:250 in blocking buffer for 48 h at 4 °C. The following antibodies were used in this paper: anti-ASY1 antibody [29] , anti-RAD51 (ref. 30 ) and anti-MLH1 (ref. 31 ) all raised in rabbit, and anti-ZYP1 (ref. 32 ) raised in guinea pig. Pads were washed for 3 h (6 × 30 min) in PBS, 0.1% Tween 20, 1 mM EDTA pH 8 and incubated for 2 h at room temperature with the appropriate secondary antibody diluted 1:200 in blocking buffer (Alexa Fluor 488 anti-rabbit antibody and Alexa Fluor 633 anti-guinea pig, Molecular Probes). The pads were washed for 3 h (6 × 30 min) in PBS, 0.1% Tween 20, 1 mM EDTA pH 8 followed by a 15 min wash in PBS. DAPI at 1 μg ml −1 was applied on the pads for 3 min and washed in PBS for 15 min. The pads were mounted in Prolong Gold antifade reagent (Molecular Probes) and left to cure for 2 or 3 days (to reach an optimum 1.47 refractive index) before being sealed with nail varnish. Image acquisition and analysis Nuclei were optically sectioned using a Leica TCS SP5II confocal laser scanning microscope controlled by Leica LAS-AF software. Z-stacks were deconvolved using AutoQuant X2 (Media Cybernetics). Projections and analysis of 3D pictures were performed using Fiji (an implementation of ImageJ, a public domain program by W. Rasband available from http://rsb.info.nih.gov/ij/ ). More than 300 nuclei obtained from multiple wheat and wheat–rye hybrid plants were scored by this method. Some of these nuclei were then selected for further analysis using Imaris 7.6.5 (Bitplane). Imaris allows the Z-stacks to be rendered in 3D; following this, the bivalents were traced by 3D modelling. The selection of MHL1 sites was performed automatically using the ‘spot detection’ wizard in Imaris 7.6.5, and the results were subsequently manually edited to remove any sites that lay away from the nucleus or to add in sites that the automatic detection failed to select. Statistical analysis Student’s t -test was performed using GenStat 16th edition (VSN International Ltd, UK). Tests are two-sided, and a P -value of 0.05 was set to be statistically significant. How to cite this article: Martín, A. C. et al. Licensing MLH1 sites for crossover during meiosis. Nat. Commun. 5:4580 doi: 10.1038/ncomms5580 (2014).